Ocean currents generate large footprints in marine palaeoclimate proxies Fossils of marine microorganisms such as planktic foraminifera are among the cornerstones of palaeoclimatological studies. It is often assumed that the proxies derived from their shells represent ocean conditions above the location where they were deposited. Planktic foraminifera, however, are carried by ocean currents and, depending on the life traits of the species, potentially incorporate distant ocean conditions. Here we use high-resolution ocean models to assess the footprint of planktic foraminifera and validate our method with proxy analyses from two locations. Results show that foraminifera, and thus recorded palaeoclimatic conditions, may originate from areas up to several thousands of kilometres away, reflecting an ocean state significantly different from the core site. In the eastern equatorial regions and the western boundary current extensions, the offset may reach 1.5 °C for species living for a month and 3.0 °C for longer-living species. Oceanic transport hence appears to be a crucial aspect in the interpretation of proxy signals. Marine sediment archives have been paramount in forming our understanding of centennial- to orbital-scale climate and environmental change [1] , [2] , [3] , [4] , [5] . Much of the palaeoclimatic information has been obtained from the geochemistry of fossil planktic foraminifer shells and from their species assemblage composition. It has been known for a long time that the drift of planktic foraminifera may mean they record water conditions different from conditions at the core site [6] . The influence of the provenance of foraminifera on proxy signals during their life cycle, however, has not been assessed and quantified in a rigorous manner, using high-resolution ocean models. Besides the fact that planktic foraminifera employ a mechanism to control their depth habitat [7] , they can be considered as passive particles, sensitive to advective processes by ocean currents. As they grow their calcite shell during their lifespan, foraminifera may drift across different climate zones and ocean regimes. At the end of their life cycle—during the phase of gametogenesis—foraminifera lose their ability to stay buoyant in the upper ocean and their shells sink to the ocean floor to become part of the sedimentary geological archive [1] , [2] , [3] , [4] , [5] , [8] . Although the horizontal advection distance for post-mortem sinking foraminifera has been estimated at a few hundred kilometres [6] , [9] , [10] , [11] , [12] , there is a remarkable dearth of information on the geographical footprint of foraminifera during their lifespan. Here we quantify the lateral distance that planktic foraminifera can cover during their lifespan and quantify the impact of the ambient temperature along their trajectory on the signal incorporated into their shells. We show that this impact is potentially highly significant in regions of fast-flowing surface currents such as western boundary currents. To illustrate the impact of the trajectory integrated temperature signal during life and transport on the proxy, we focus on the Agulhas region, where planktic foraminifera have been extensively used to study variations and global influence of the amount of warm tropical Indian Ocean water flowing into the Atlantic Ocean [5] , [13] , [14] . Foraminiferal traits and their relation to drift We use two ocean models of contemporary circulation, which both include mesoscale eddies, to study the advection during the life span and the post-mortem sinking of foraminifera. Both models have a 1/10° horizontal resolution, but their domains differ: the INALT01 model [15] is focused around southern Africa in the Agulhas system and is among the best-performing models in that region [13] , [15] , [16] , [17] , while the Ocean model For the Earth Simulator (OFES) model [18] is global in extent, allowing us to place these results in a wider context. In both models, we advect the virtual foraminifera as passive Lagrangian particles using the Connectivity Modeling System (CMS) [19] , simulating both their trajectories during their lifetime, as well as their post-mortem sinking. The local in situ temperature from the hydrodynamic models is interpolated onto the particle trajectories and used to reconstruct the incorporation of the temperature signal during the virtual foraminifera’s lifetime. We compare the model results to combined single-shell δ 18 O and multiple-shell Mg/Ca temperature reconstructions from Globigerinoides ruber from core tops at two locations in the Agulhas region [1] : (1) site CD154-18-13P below the Agulhas Current and (2) site MD02-2594 below the Agulhas leakage area. Foraminifer traits such as depth habitat, lifespan, seasonality, post-mortem sinking speed and rate of growth (which is related to rate of calcification) vary widely between species and are often poorly constrained [6] , [8] , [20] , [21] . Focusing on surface-dwelling foraminifera, we therefore undertook a sensitivity assessment of these different traits. Values for sinking speed employed in the models were 100, 200 and 500 m per day and depth habitats were 30 and 50 m. Lifespans were related to the synodic lunar cycle [8] , [20] , with 15 days for G. ruber and 30 days for other surface-dwelling foraminifera. However, as some studies report even longer life spans for upper water column dwelling foraminifera [6] , [20] , we also investigated extended lifespans of 45 days within the INALT01 model and 180 days within the global OFES model. Two growth rates were used to simulate different calcification scenarios. One was a linear growth scenario, where the recorded calcification temperature of a virtual foraminifer is the mean temperature along its trajectory during its lifespan. The other was an exponential growth scenario, with a growth rate [7] , [22] of 0.1 per day, so that the later life stages of the foraminifera weigh more heavily in the final calcification temperature [8] , [23] . Finally, we studied the effect of a seasonal growth cycle on the recorded temperatures. See Methods section for further methodological information. Foraminifera drift in the Agulhas region A substantial fraction of the particles incorporated in the cores from both the Agulhas Current and the Agulhas leakage region appears to originate from hundreds of kilometres away ( Fig. 1 ). Using a depth habitat of 50 m, a lifespan of 30 days and a sinking speed of 200 m per day, the average drift distances, which are defined as the average shortest distance from spawning location to the core site for all virtual foraminifera, are 713 and 533 km in the Agulhas Current and Agulhas leakage, respectively. These distances are more than four times larger than the drift distances during their post-mortem sinking (which are 166 and 71 km for the Agulhas Current and Agulhas leakage, respectively, Fig. 2a,b ), highlighting the impact of drift during the virtual foraminifer’s life. 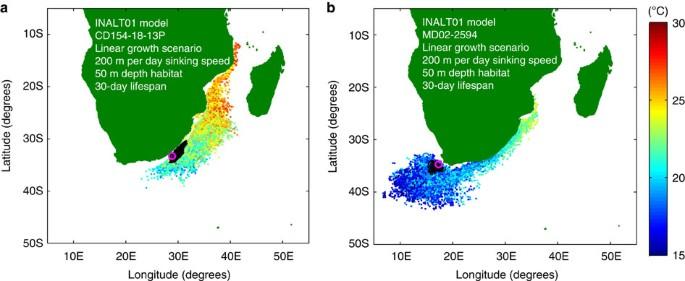Figure 1: Foraminifera footprints in the Agulhas region. Maps of the footprint for two core sites in (a) the Agulhas Current and (b) the Agulhas leakage region. Each coloured dot represents the location where a virtual foraminifer starts its 30-day life, colour-coded for the recorded temperature along its trajectory. Black dots represent where foraminifera die and start sinking to the bottom of the ocean (at 200 m per day) to end up at the core location (indicated by the purple circle). Figure 1: Foraminifera footprints in the Agulhas region. Maps of the footprint for two core sites in ( a ) the Agulhas Current and ( b ) the Agulhas leakage region. Each coloured dot represents the location where a virtual foraminifer starts its 30-day life, colour-coded for the recorded temperature along its trajectory. Black dots represent where foraminifera die and start sinking to the bottom of the ocean (at 200 m per day) to end up at the core location (indicated by the purple circle). 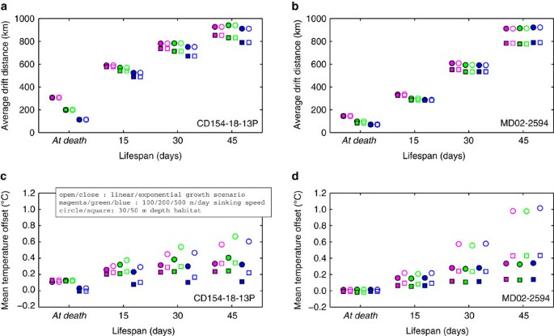Figure 2: The dependence of foraminifera footprint on life traits. The sensitivity of the chosen foraminiferal traits on (a,b) the average distance between spawning and core location, and on (c,d) the offset between the mean recorded temperature and the local temperature at the two core sites depicted in Fig. 1. Lifespan is on thexaxis, with ‘at death’ the assumption that foraminifera record the temperature of the location in the last day before they die and start sinking. The results depend noticeably on the traits, except for the sinking speed (colours), which seems to have little effect on mean recorded temperature. Full size image Figure 2: The dependence of foraminifera footprint on life traits. The sensitivity of the chosen foraminiferal traits on ( a , b ) the average distance between spawning and core location, and on ( c , d ) the offset between the mean recorded temperature and the local temperature at the two core sites depicted in Fig. 1. Lifespan is on the x axis, with ‘at death’ the assumption that foraminifera record the temperature of the location in the last day before they die and start sinking. The results depend noticeably on the traits, except for the sinking speed (colours), which seems to have little effect on mean recorded temperature. Full size image This surface drift has implications for the recorded temperature. In the case of the Agulhas Current core ( Fig. 1a ), some of the virtual foraminifera start their life in the Mozambique Channel and the temperature recorded by these specimens along their 30-day life is up to 5 °C warmer than at the core site. Such an offset is much larger than the uncertainty of 1.5 °C (2 σ ) that is associated with foraminifera proxy-based temperature reconstructions [9] , [10] , [11] , [24] . In the core at the Agulhas leakage region ( Fig. 1b ), some particles arrive from warmer subtropical temperature regimes of the northern Agulhas Current, whereas others—in our model—originate from the sub-Antarctic cold waters of the Southern Ocean in the south. Both the average drift distances as well as the recorded temperatures are strongly dependent on the values chosen for the foraminifer traits ( Fig. 2 ). The dependence is nonlinear and different for the two sites, although general patterns emerge: sinking speed is the least important trait; growth scenario becomes more important for longer-living foraminifera; depth habitat has far less effect on drift distance than on recorded temperature ( Supplementary Figs 1–4 ). There are also differences between the INALT01 and the OFES models, particularly in the amount of virtual foraminifera originating far upstream in the Agulhas Current, which show the dependency of the results on the circulation state ( Supplementary Fig. 5 ). However, there does not seem to be a seasonal variation in the temperature offsets ( Fig. 3 ). 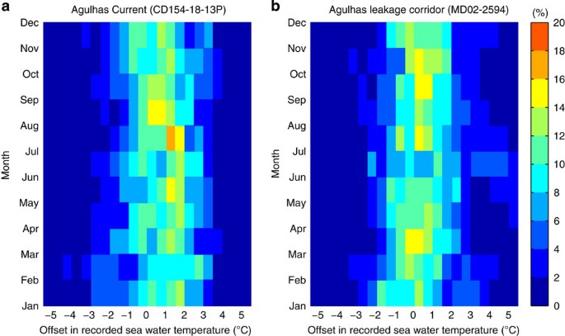Figure 3: The effect of seasonality on the temperature offsets. Seasonal cycle of the offset of recorded temperature for the virtual foraminifera with respect to the localin-situtemperature in (a) the Agulhas Current core and (b) the Agulhas leakage core. For each month, the difference between the recorded temperatures and the instantaneous temperatures at the core is plotted with a 0.5 °C interval, as a percentage of the total number of virtual foraminifera that reach the core in that month. The virtual foraminifera have a lifespan of 30 days, a depth habitat of 50 m, a linear growth scenario and a sinking speed of 200 m per day. There is no clear seasonal variation in offset of recorded temperatures with time of year. Figure 3: The effect of seasonality on the temperature offsets. Seasonal cycle of the offset of recorded temperature for the virtual foraminifera with respect to the local in-situ temperature in ( a ) the Agulhas Current core and ( b ) the Agulhas leakage core. For each month, the difference between the recorded temperatures and the instantaneous temperatures at the core is plotted with a 0.5 °C interval, as a percentage of the total number of virtual foraminifera that reach the core in that month. The virtual foraminifera have a lifespan of 30 days, a depth habitat of 50 m, a linear growth scenario and a sinking speed of 200 m per day. There is no clear seasonal variation in offset of recorded temperatures with time of year. Full size image The distribution of the calcification temperatures of the virtual foraminifera can be compared with proxy temperature distributions derived from the G. ruber from the core tops (see Methods). The mean±1 s.d. of the INALT01, OFES and proxy distributions overlap ( Fig. 4 ). The spread in temperatures is larger than the typical sensitivities to the choice of life trait values (which is <1 °C, Fig. 2c,d ). According to a two-sample Kolmogorov–Smirnov test, the G. ruber proxy data in the Agulhas Current core is most closely matched by the virtual foraminifera within OFES with a depth habitat of 30 m ( P =0.47, which means the OFES and proxy distributions are statistically indistinguishable). The G. ruber proxy data in the Agulhas leakage core is most closely matched by the virtual foraminifera within INALT01, with a depth habitat of 50 m ( P =0.06). All other virtual foraminifera distributions are statistically different from the G. ruber proxy data ( P <0.05), even though in all cases means and s.d. are within 1.5 °C of the G. ruber proxy data. 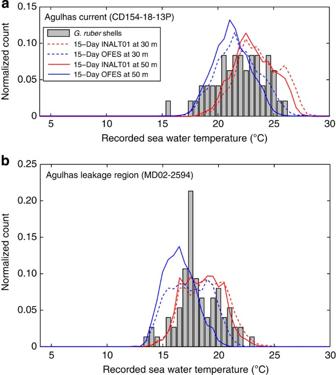Figure 4: Distributions of temperature at two cores in the Agulhas region. The observed proxy temperatures (grey bars) at (a) the Agulhas Current core and (b) the Agulhas leakage core are compared with the temperature distributions for the virtual foraminifera experiments in the INALT01 model (red) and the OFES model (blue). Traits used are theG. ruberlifespan20of 15 days, a depth habitat of 30 m (dashed) or 50 m (solid), a sinking speed of 200 m per day and a linear growth scenario. Note that the spread in recorded temperature is larger than the sensitivity of the means with foraminiferal trait choices (Fig. 2c,d). Figure 4: Distributions of temperature at two cores in the Agulhas region. The observed proxy temperatures (grey bars) at ( a ) the Agulhas Current core and ( b ) the Agulhas leakage core are compared with the temperature distributions for the virtual foraminifera experiments in the INALT01 model (red) and the OFES model (blue). Traits used are the G. ruber lifespan [20] of 15 days, a depth habitat of 30 m (dashed) or 50 m (solid), a sinking speed of 200 m per day and a linear growth scenario. Note that the spread in recorded temperature is larger than the sensitivity of the means with foraminiferal trait choices (Fig. 2c,d). Full size image A global estimate of foraminifera drift A global analysis ( Fig. 5 ), using the OFES model, of virtual foraminifera released on a 5° × 5° global grid reveals that the virtual foraminifera can drift for up to a thousand kilometres during an assumed 30-day lifespan ( Fig. 5c ). This is one order of magnitude larger than the lateral drift, which dead virtual foraminifera experience during the 200 m per day sinking ( Fig. 5a ). Drifts are largest in regions with largest horizontal velocities such as along the equator, in the western boundary currents and their extensions, and in the Southern Ocean, while drift distances are smaller in the centres of the gyres. 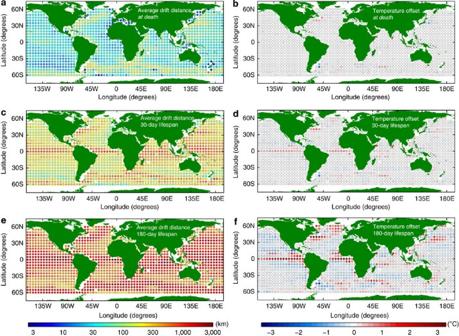Figure 5: Global analysis of drift distances and temperature offsets. (a,c,e) The average distance between spawning location and the core site for virtual foraminifera in the OFES model that record the temperature (a) in the last day before they die and start sinking and for virtual foraminifera with lifespans of (c) 30 days and (e) 180 days. In all cases, a depth habitat of 50 m, a linear growth scenario and a sinking speed of 200 m per day were used. Note that the colour scale is logarithmic. (b,d,f) Offsets, defined as the difference between along-trajectory recorded temperatures and local temperatures at the core site. Offsets reach up to 1.5 °C for 30-day lifespans and up to 3 °C for 180-day lifespans, when the virtual foraminifera travel more than 1,000 km. Figure 5: Global analysis of drift distances and temperature offsets. ( a , c , e ) The average distance between spawning location and the core site for virtual foraminifera in the OFES model that record the temperature ( a ) in the last day before they die and start sinking and for virtual foraminifera with lifespans of ( c ) 30 days and ( e ) 180 days. In all cases, a depth habitat of 50 m, a linear growth scenario and a sinking speed of 200 m per day were used. Note that the colour scale is logarithmic. ( b , d , f ) Offsets, defined as the difference between along-trajectory recorded temperatures and local temperatures at the core site. Offsets reach up to 1.5 °C for 30-day lifespans and up to 3 °C for 180-day lifespans, when the virtual foraminifera travel more than 1,000 km. Full size image This horizontal drift can introduce large offsets when foraminiferal records are interpreted as representative of local conditions: for example, in the reconstruction of temperatures, the discrepancy with the local temperatures varies greatly with region ( Fig. 5b,d,f ). If it is assumed that the foraminifera document the local temperature at the location where they die and start sinking, the offsets are smaller than 0.1 °C almost everywhere ( Fig. 5b ). However, for lifespans of 30 days [6] , [20] , offsets can be as large as 1.5 °C ( Fig. 5d ), which is equal to the uncertainty associated with proxy-based palaeotemperature estimates [9] , [10] , [11] , [24] . Virtual G. ruber , with lifespans of 15 days, have similar offsets ( Supplementary Fig. 6 ). For virtual foraminifera with more extended lifespans of 180 days ( Fig. 5e,f ), average drift distances can reach 3,000 km and the associated offsets in average recorded temperature can be >3 °C. In the case of virtual foraminifera with depth habitats of 30 m, these temperature offsets are up to 4 °C ( Supplementary Fig. 7 ), while they are up to 2 °C in the case of an exponential growth scenario ( Supplementary Fig. 8 ). We have shown that ocean currents affect the signals incorporated in foraminiferal proxies. There appears to be a clear global pattern in the global temperature offsets, which are positive along the equator and within the western boundary currents, and negative in the centres of the subtropical gyres. The regions with largest temperature offsets are those closely related to regions of high ocean surface velocity and consequently lateral drift: in the eastern Tropical Pacific and Atlantic Ocean, and in the extensions of the western boundary currents such as the Gulf Stream, Kuroshio and Agulhas currents. However, there are also regions of high lateral drift where temperature offsets are much smaller such as the Southern Ocean and the Tropical Indian Ocean. The difference is that the regions of high offsets are also the regions of some of the largest lateral temperature gradients (often related to large ocean–atmosphere heat fluxes). Larger temperature changes experienced by the foraminifera along their pathway result in larger offsets with respect to the temperature above the core site. The implication is that, depending on species traits and locations, the temperature offsets can be significant if the shells in the core are interpreted as representative of the conditions right above the core location. An analysis such as the one presented here could also be used a priori to identify the amount of advective bias at a potential drilling site. Another tantalizing application could be to ‘invert’ the problem and use our approach to determine where different fossil specimens most probably grew their shell, so that the temperatures recorded by the fossils could be geolocated to the location where the microorganism actually grew its shell, rather than where it reached the ocean floor. This would allow disentanglement of proxy data from microorganisms with different traits and a better spatial interpretation of the signal around the location of the sediment core site. Coccolithophores, for example, are also paleoclimatological proxy carriers of primary importance, with life traits and settling dynamics that differ notably from planktic foraminifera [25] . With an approach similar to ours, coccolithophoric footprints could be calculated and compared with the foraminiferal ones, potentially vastly increasing the amount of information that can be obtained from a single sediment core. A vital prerequisite to this application, however, is a better understanding and quantification of the organism’s ecology [20] , [26] , including species-specific lifespans, depth habitats, calcification rates and sinking speeds. Ocean model data We used data from two ocean circulation models. The first is the INALT01 model configuration [15] , which is based on the NEMO ocean model [27] , extending an earlier setup [16] . The model was specifically set up to study the dynamics of the Agulhas region and includes a 1/10° high-resolution region with 46 vertical levels that spans the entire South Atlantic and western part of the Southern Indian (between 70°W–70°E and 50°S–8°N), which is nested in a 1/2° global model. We used 28 years (1980–2007) of the hindcast experiment, a period for which the dynamics of the model has been shown to agree well with observations [15] , [16] . The atmospheric forcing builds on the CORE reanalysis products [28] and is applied via bulk air–sea flux formulae. We used the same 28 years of data from the Japanese OFES [18] , which is also 1/10° horizontal resolution and has a near-global coverage between 75°S and 75°N, and 53 vertical levels. The model is forced using National Centers for Environmental Prediction (NCEP) wind and flux fields. Results from both models have been shown to be consistent with important observed features of the modern ocean circulation, including among others the trajectories of surface buoys [29] and the deep currents in the North Atlantic [30] , the South Atlantic [31] and the Agulhas region [17] , [32] . Virtual foraminifera trajectory calculations The virtual foraminifera were advected within the INALT01 and OFES velocity data using the CMS version 1.1b [19] . The CMS employs a fourth-order Runge–Kutta method and can output along-trajectory temperature and salinity. For each core, we computed Lagrangian particle trajectories in reverse time. We started one particle every day at the core site itself, near the ocean floor, for a total of almost 10,000 particles per site (amounting to 27 simulated years). These particles were then integrated backwards in time by reversing the sign of the velocity components. A sinking velocity was added to the particles. Once near the surface, the particles were advected for another 45 days (180 days in the global case) at their prescribed depth habitat, using only the horizontal velocity fields and without any explicit diffusivity (see below). During this part of their trajectory, representing the lifespan of the foraminifera, the location as well as the in situ temperature of the particle was stored every day for further analysis. These along-trajectory temperatures were then used to offline calculate the recorded temperature based on growth scenario. The temperature distributions along the trajectory paths were then compared with in situ conditions at the core location. For sites poleward of 40°N and 40°S in the global experiment, we used only those virtual foraminifera that lived for their full life in the warmer months (April to September for the Northern Hemisphere and October to March for the Southern Hemisphere). In all other cases, including those of the Agulhas region cores, we used virtual foraminifera throughout the year and have not observed a bias in the results that would be associated with seasonality ( Fig. 3 ). Sensitivity to the addition of diffusion in foraminiferal transport The particles in this study have been computed using the three-dimensional model velocity fields, without any additional diffusion due to sub-grid scale processes. Here we show that the effect of diffusion is an order of magnitude smaller than that of advection with the currents ( Supplementary Fig. 9 ). In these simulations, we used the turbulent diffusion module of the CMS (equation 3 in ref. 19 ) with K h =50 m 2 s −1 for the MD02-2594 core and with K h =250 m 2 s −1 for the CD154-18-13P core. We chose the first of these values for diffusion ( K h =50 m 2 s −1 ) as the most appropriate for the INALT01 and OFES models, which both have a resolved scale of 10 km (Fig. 2 of ref. 33 ). The second of these values ( K h =250 m 2 s −1 ) was chosen to study the effect of an extremely high diffusivity. The experiments revealed that for both cores, the effect of diffusion on the core footprints is minimal. In the case of core MD02-2594, the average shortest distance between spawning location and core site changed by only 10 km. In the case of core CD154-18-13P, which had the much higher diffusivity, the average distance changed only by 18 km. This finding is in agreement with previous results where it was shown (Fig. 1 of ref. 33 ) that diffusion on time scales of months is <50 km. It is also in agreement with the theoretical estimate of dispersion in the absence of advective flow. A Brownian motion process gives for the spread of particles std( X )=sqrt(2 K h T ), where std( X ) is the s.d. of distance (that is, the spread due to diffusion) and T is the length of integration. For T =30 days and K h =50 m 2 s −1 this leads to std( X )=16 km, whereas for the longer OFES runs with T =180 days and K h =50 m 2 s −1 this leads to std( X )=40 km. In summary, diffusivity in the 1/10° resolution OFES and INALT01 models is at least an order of magnitude smaller than the advective spread we find in our study, and hence diffusion will not affect our main conclusions. Literature review of the sinking speed of planktic foraminifera We consider a set of surface-dwelling planktic foraminifer species, widely used to reconstruct sea surface conditions such as temperatures. The depth habitat of these species can be confidently constrained to the mixed layer, therefore warranting the assumption that no significant vertical migration during living time occurs [8] , [20] . We reviewed the specialized literature for the most accurate quantification of the sinking speed of foraminifera shells ( Table 1 ). The results of previous studies (see references in Table 1 ) confirm that the sinking speed of planktic foraminifera depends mainly on the shell weight (in turn related to the shell size, that is, diameter) and the presence of spines. From the same studies, it appears that the shell morphology, which is characteristic of each species, is also determinant for the sinking speed. Shell thickening is also important and it is related to the life stage of the specimen, which in turn is arguably proportional to the shell size. Table 1 Values of sinking speeds retrieved from laboratory studies. Full size table Therefore, following ref. 21 , we chose to use a sinking speed of 200 m per day for non-ashed G. ruber with a common size of ~300 μm. This was based on four considerations: first, G. ruber , Globigerinoides sacculifer and Globigerinoides bulloides are among the most used surface foraminifer species in palaeo-reconstructions; second, foraminifera in the size fraction between 200 and 350 μm are the most used; third, even though foraminifera might undergo partial post-mortem degradation of their plasma content, and although before sinking they normally release their gametes, which constitute a large part of their organic composition, the non-ashed, plankton-tow sample probably resembles the form in which a foraminifer sinks just after death; and finally, seawater (as opposed to freshwater) experiments more closely mime the dynamics of foraminifera sinking. Empirical data from G. ruber shells Shells of planktic foraminifer G. ruber , white variety, were picked from the top centimetre of cores MD02-2594 (Agulhas leakage region, 34° 42.6′ S, 17° 20.3′ E, 2,440 m depth) and CD154-18-13P (Agulhas Current, 33° 18.3′ S, 28° 50.8′ E, 3,090 m depth), from the size fraction 250–355 μm. Both core tops represent contemporary climate (see below). Stable isotope (δ 18 O) analyses were conducted on the single shells with a Thermo Finnigan Delta Plus mass spectrometer at the VU University Amsterdam, with the method outlined in ref. 13 . We analysed 79 G. ruber shells from core MD02-2594 and 48 shells from core CD154-18-13P. From core MD02-2594, we also analysed the Mg/Ca value of a group of 20 shells of G. ruber , using an inductively coupled plasma/optical emission spectrometry, after rigorous cleaning of the sample, following a standard procedure [34] . Analysis was performed at the Trace Elements Laboratory of Uni Research, Bergen. As for core CD154-18-13P the amount of shells did not allow carrying out Mg/Ca analysis, we used the Mg/Ca value of the core top of adjacent core CD154-17-17K (33° 16.1′ S, 29° 7.3′ E, 3,330 m depth) [14] , which is located 26 km to the SE. Temperature reconstructions from G. ruber geochemistry The Mg/Ca values were converted to calcification temperatures using a species-specific calibration [24] . We used a previously established approach to assign calcification temperatures to individual foraminiferal shell [2] , which consists of first anchoring the mean temperature of the foraminiferal population using the Mg/Ca-derived temperature of a group of shells; then calculating the offset of each shell δ 18 O value from the mean of all measurements; and finally converting each δ 18 O offset into a temperature offset by dividing it by a factor of −0.22, which approximates the dependency of equilibrium calcite δ 18 O eq on temperature [35] . This method necessarily assumes that only temperature determines the foraminiferal δ 18 O (δ 18 O f ), thus ignoring a potential effect of changes in seawater δ 18 O (δ 18 O w ) that can be measurable near ocean fronts [36] such as the subtropical front near 40°S south of Africa. Given the northerly location of our Agulhas leakage core at 34°S, this is not a major concern for our study and we consider this approach to yield a reasonable first-order approximation of palaeo upper water column temperature variability from a foraminiferal population as previously shown [2] . Radiocarbon dating of the core tops One assumption in the comparison between palaeo proxy data and INALT01 model ( Fig. 4 ) is that the two core tops are representative of the same contemporary circulation as the model. We support the validity of this assumption in the following. Core MD02-2594 in the Agulhas leakage area has been dated at a depth of 50–51 cm, to be 2,815±57 years before present [37] . Therefore, the core top itself will be younger than that. Core CD154-18-13P in the Agulhas Current has not been radiocarbon dated, but the core top of core CD154-17-17K, <50 km away, has been dated at a calibrated age of between 1,760 and 1,849 years before present [38] . As a further confirmation that the core top material of CD154-18-13P is representative at least of the Holocene, we verify that the average δ 18 O value of the core top G. ruber specimens we analysed (−1.29±0.5‰; error is s.d. of 48 measurements) is comparable—if not more negative—to that of CD154-17-17K core top (−1.13±0.1‰; error is instrument precision [38] ). A radiocarbon date on CD154-18-13P core top should be obtained to certify this, but this was not possible due to scarcity of material. In summary, both core tops are of at least Late Holocene age, which suggests that our foraminiferal analyses should reflect the dynamics and ocean properties of the modern Agulhas System. How to cite this article: van Sebille, E. et al . Ocean currents generate large footprints in marine palaeoclimate proxies. Nat. Commun. 6:6521 doi: 10.1038/ncomms7521 (2015).